Ionization of Rydberg atoms by standing-wave light fields When electromagnetic radiation induces atomic transitions, the size of the atom is usually much smaller than the wavelength of the radiation, allowing the spatial variation of the radiation field’s phase to be neglected in the description of transition rates. Somewhat unexpectedly, this approximation, known as the electric dipole approximation, is still valid for the ionization of micrometre-sized atoms in highly excited Rydberg states by laser light with a wavelength of about the same size. Here we employ a standing-wave laser field as a spatially resolving probe within the volume of a Rydberg atom to show that the photoionization process only occurs near the nucleus, within a volume that is small with respect to both the atom and the laser wavelength. This evidence resolves the apparent inconsistency of the electric dipole approximation’s validity for photoionization of Rydberg atoms, and it verifies the theory of light–matter interaction in a limiting case. The electric dipole approximation is at the heart of perturbative atomic photoionization studies at low intensity [1] . To understand the approximation’s boundaries, it is important to explore cases in which one might expect it to break down. In the extreme case of soft X-rays interacting with ground-state atoms (sizes ~10 −10 m), experiments have demonstrated non-dipole photoemission patterns [2] . A complementary extreme case occurs in the interaction of Rydberg atoms with light fields (atom size~wavelength~10 −6 m). Despite the apparent violation of the dipole approximation in this case, photoionization rates agree with calculated rates based on the approximation. For example, measured photoionization rates for various nD 5/2 states of Cs Rydberg atoms in an approximately homogeneous 1,064 nm field are in agreement with calculations that make the approximation [3] . To reconcile this apparent inconsistency, one may argue that the photoionization process occurs close to the nucleus in the atom [4] , [5] , [6] . This argument has been utilized in previous Rydberg-atom wave packet experiments to probe the probability of the wave packet return to the nucleus [7] , [8] . However, the argument has never been directly verified with a photoionization probe that has sub-atomic spatial resolution. Here, we investigate the photoionization process as a function of position within the volume of a Rydberg atom. We employ 85 Rb Rydberg nD levels in a one-dimensional optical standing wave, formed by a pair of counter-propagating laser beams of wavelength 1,064 nm. Laser beam intensities are on the order of 10 8 W cm −2 , which is low enough that higher order effects such as above-threshold ionization do not occur, and photoionization rates scale proportionally to intensity. The extent of the Rydberg electronic wavefunction approximately equals the standing-wave period, which results in maximal intensity contrast of the light field within the volume of the atom. 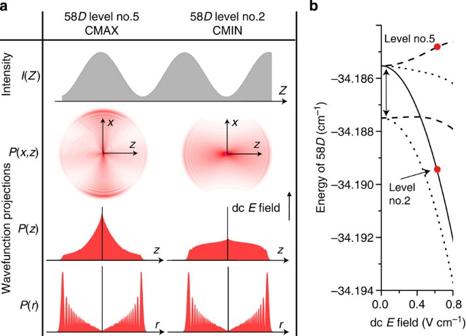Figure 1: 58Dstates in an optical standing wave and d.c. electric field. (a) The standing-wave intensity,I(Z), and projections of the electron probability density in the (xz)-plane, thez-coordinate and the radialr-coordinate. Lowercase letters, relative coordinates of the Rydberg electron; uppercase letters, centre-of-mass coordinates. Atoms prepared with initial condition CMAX (CMIN) have centre-of-mass positions located near intensity maxima (minima). (b) Stark energy level diagram. The fine structure splitting at zero electric field (double-headed arrow) is 60 MHz. Electric fields and energies for the projections are indicated by circles. Solid line: |mj|=5/2. Dotted lines: |mj|=3/2. Dashed lines: |mj|=1/2. Figure 1a illustrates the relation between the wavefunctions and the optical standing wave for two of the states that we examine. The antinodes of the standing wave are placed either near the atom’s centre or within the main lobes of the electronic probability distribution. The measured photoionization rates under these contrasting conditions indicate whether it is the light-field intensity near the centre of the atom or within the lobes of the electronic probability distribution that matters in the photoionization process. Although intuition might suggest that photoionization occurs where the probability of finding the electron is greatest, we demonstrate in this work that the process in fact happens near the nucleus. Figure 1: 58 D states in an optical standing wave and d.c. electric field. ( a ) The standing-wave intensity, I ( Z ), and projections of the electron probability density in the ( xz )-plane, the z -coordinate and the radial r -coordinate. Lowercase letters, relative coordinates of the Rydberg electron; uppercase letters, centre-of-mass coordinates. Atoms prepared with initial condition CMAX (CMIN) have centre-of-mass positions located near intensity maxima (minima). ( b ) Stark energy level diagram. The fine structure splitting at zero electric field (double-headed arrow) is 60 MHz. Electric fields and energies for the projections are indicated by circles. Solid line: | m j |=5/2. Dotted lines: | m j |=3/2. Dashed lines: | m j |=1/2. Full size image Experimental set-up 85 Rb ground-state atoms are collected in a magneto-optical trap with a temperature of ~150 μK and then loaded into a one-dimensional optical standing wave formed by counter-propagating 1,064 nm laser beams (referred to as an optical lattice). Ground-state atoms are transferred to Rydberg states (45≤ n ≤65) via two-photon excitation (Methods). The number of Rydberg atoms is determined by ionizing them with an electric field pulse [9] and detecting the freed electrons with a microchannel-plate assembly. The Rydberg atoms are prepared in the optical lattice with initial centre-of-mass positions either near intensity maxima, which we refer to as initial condition CMAX, or near intensity minima, referred to as initial condition CMIN (Methods). For condition CMAX, the electronic probability distributions are predominately peaked near intensity minima, whereas for condition CMIN, they predominately peak near intensity maxima. A comparison of photoionization for these two conditions reveals whether it is the light-field intensity near the atom’s nucleus or within the lobes of the electronic probability distribution that determines the photoionization rates. To establish well-defined electronic probability distributions in the optical lattice with which to probe the photoionization behaviour, we apply a d.c. electric field ( Fig. 1 ), oriented transverse to the lattice axis. The Stark effect lifts the degeneracy of the | m j | sublevels of the Rydberg nD states. As shown in Fig. 1b , the frequency of the excitation lasers is chosen to excite the Rydberg levels no. 2 or no. 5 within the Stark nD manifolds. We choose these levels because their electronic probability distributions with respect to the lattice are quite different, to test whether such differences influence the photoionization behaviour. In Fig. 1a , we display projections of the electron density, P ( x , z ) and P ( z ), as well as the radial probability distribution, P ( r ), where x , z and r are relative coordinates of the Rydberg electron. In our experiment, we aim to demonstrate whether the photoionization rate is dependent on the overlap ∬ P ( z ) I ( z + Z )d z of the electron with the lattice intensity I , or whether it only depends on the intensity at the centre-of-mass location Z and the probability of finding the electron close to the nucleus (that is, within a small central region of P ( r )). Measurement procedure We determine the photoionization rate ( γ PI ) of a Rydberg level from measurements of its decay rate within the lattice (which yields the sum of radiative, blackbody and photoionization decay rates, γ rad + γ bb + γ PI ) and without the lattice (which yields γ rad + γ bb ). By subtracting the lattice-free decay rate from that within the lattice, we obtain a measurement of γ PI . We measure a level’s decay rate by recording the number of Rydberg atoms as a function of t d , the delay time between the end of the excitation pulse and detection. The number of Rydberg atoms excited per cycle is only 1–2, ensuring that interactions and collisions between Rydberg atoms have no role. To determine the lattice-free decay rate of a level, the number of atoms is measured for 0≤ t d ≤60 μs ( n =45) and 0≤ t d ≤150 μs ( n =50, 58 and 65). The data are fit to an exponential; the fit yields the lattice-free decay rate ( γ rad + γ bb ) :=1/ τ o . An example of lattice-free decay data is shown in Fig. 2a,b (circles). Our measured values of τ o , found in Table 1 , are consistent with our calculations for a 77 K environment (our set-up) and with values found elsewhere [10] , [11] . 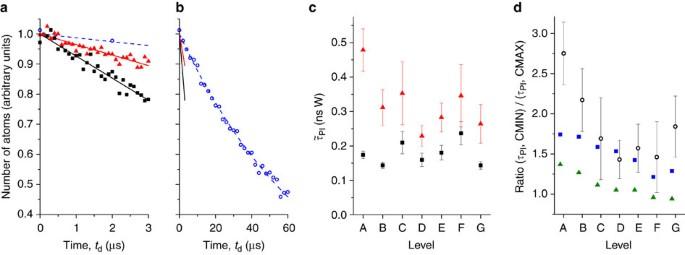Figure 2: Photoionization of Rydberg atoms in an optical lattice. (a,b) Example of measured atom number versus time for 45Dlevel no. 5. Decay rates are determined from fits. Solid symbols and linear fits: lattice present; atom centre-of-mass positions with initial conditions CMAX (squares) and CMIN (triangles). Hollow circles and dashed exponential fit: without lattice. (c) Normalized photoionization lifetimes,with effective quantum numbern* and lattice powers from Table 1, for CMAX (squares) and CMIN (triangles). Level labels explained inTable 1. The lifetimes are an average of 1,000 (levels A, B and E), 1,250 (D and F) and 1,750 (C and G) measurements. Error bars represent the standard error of the mean, s.e.m. (d) Ratios of photoionization lifetimes for initial condition CMIN to those with initial condition CMAX. Circles: experimental. Error bars, s.e.m. Squares: calculated, using equation (1). Triangles: calculated, using comparison model. Figure 2: Photoionization of Rydberg atoms in an optical lattice. ( a , b ) Example of measured atom number versus time for 45 D level no. 5. Decay rates are determined from fits. Solid symbols and linear fits: lattice present; atom centre-of-mass positions with initial conditions CMAX (squares) and CMIN (triangles). Hollow circles and dashed exponential fit: without lattice. ( c ) Normalized photoionization lifetimes, with effective quantum number n * and lattice powers from Table 1, for CMAX (squares) and CMIN (triangles). Level labels explained in Table 1 . The lifetimes are an average of 1,000 (levels A, B and E), 1,250 (D and F) and 1,750 (C and G) measurements. Error bars represent the standard error of the mean, s.e.m. ( d ) Ratios of photoionization lifetimes for initial condition CMIN to those with initial condition CMAX. Circles: experimental. Error bars, s.e.m. Squares: calculated, using equation (1). Triangles: calculated, using comparison model. Full size image Table 1 Photoionization lifetime measurement conditions and results. Full size table To determine decay rates within the lattice, the number of atoms is measured for 0≤ t d ≤3 μs. We limit t d to ≤3 μs so that the atoms spend a large fraction of the atom–field interaction time near the intensity maxima or minima where they are initially prepared (the oscillation period of the atoms in the lattice is ~5 μs). We fit the measured number of atoms as a function of t d to a line. The slope of the line divided by its y -intercept approximates the decay rate γ rad + γ bb + γ PI , averaged over the 3 μs. An example of decay data within the lattice is shown in Fig. 2a for both initial conditions CMAX (squares) and CMIN (triangles). Photoionization lifetimes The final measurement results of the photoionization lifetime τ PI =1/ γ PI for all levels are found in Fig. 2c and Table 1 . The results shown in Fig. 2c are normalized to account for the overall ( n *3 / I 1 )-scaling [12] of τ PI with ingoing beam intensity I 1 and effective principal quantum number n * ( n *= n − δ , where δ =1.35 for nD states of Rb (ref. 13 )). The normalized lifetimes are denoted by . For each level, is shorter for atom centre-of-mass positions with initial condition CMAX than for initial condition CMIN, regardless of the Rydberg electron’s probability distribution. This is true even for cases in which the main lobes of the electronic wavefunction and the atomic nucleus are separated by about half the lattice period (1,064 nm/4), a situation that maximizes the intensity contrast within the atom. This situation occurs when the atomic radius, r ≈2 n 2 , approximately equals 1,064 nm/4, corresponding to n ~50 (where most of our data is taken). Thus, a qualitative analysis of the data already demonstrates that the photoionization process depends more on the light-field intensity near the nucleus of the atom than on that within the main lobes of the electronic probability distribution. The error bars for each in Fig. 2c reflect statistical uncertainties and follow from standard error propagation and fit-parameter uncertainties returned by the fitting program (OriginPro 8). Systematic errors in the arise mainly from lattice intensity variations, originating from the lattice laser itself or from deviations in alignment of the Rydberg excitation lasers with the lattice focal spot. On the basis of our measurement procedures used for verifying the lattice depth [14] , we determine that the relative range of the lattice intensity variation is ≤8%. The effect of a reduction in lattice intensity is to move the measurements of for both initial conditions CMAX and CMIN to higher values. Model of photoionization To analyse the data quantitatively, we compute atomic trajectories from the lattice trapping potentials and simultaneously simulate the photoionization-induced decay with position-dependent γ PI . The photoionization-induced decay is simulated in two ways, chosen to reveal where the photoionization process occurs in the atom. In the first way, we employ γ PI calculated in the electric dipole approximation, γ PI = σ PI ( I ( Z ))/( ħ ω ), where I ( Z ) is the lattice light intensity at the atomic nucleus and σ PI is the photoionization cross-section [1] : M r represents the matrix element describing the coupling of the initial Stark level to the continuum (Methods). In the second way, we calculate γ PI using a comparison model in which γ PI ∝ ∬ P ( z ) I ( z + Z )d z . The decay rate in the comparison model is dominated by the light intensity in the regions where the electron probability distribution P is greatest, whereas in the model based on equation (1), it is determined by the intensity at the nucleus. In Fig. 2d , we plot the ratios of τ PI for initial condition CMIN to those for CMAX for the measurement results as well as the simulation results based on the two models of photoionization. In the simulations, we use an initial atomic temperature of 150 μK and the beam powers and focal diameters employed in the experiment. There are no other free parameters in the simulations. For a lattice with perfect contrast and for atoms frozen in place at either intensity maxima or minima, the ratio of τ PI for initial condition CMIN to that for CMAX would be infinity. On the basis of the actual contrast between intensity maxima and minima in our lattice (Methods), the maximum possible ratio that one could observe for atoms frozen in place would be about 5. Any motion of the atoms in the lattice or variations in their initial positions away from the intensity maxima or minima will further reduce the experimentally observed ratio. Comparing the simulation results for the two models of photoionization to the measurement results in Fig. 2d , we observe good agreement between the measured ratios (circles) and the model based on equation (1) (squares), which clearly gives the better account of the data than the comparison model (triangles). Quantitatively, the average deviation of the measured ratios from the calculated ratios using equation (1) is 0.11, whereas the average deviation from the comparison model is 0.26. We note that the disparities between the simulation results based on equation (1) and the experimental data for levels A, B and G can be resolved by assuming a lower atom temperature (which generally increases the contrast between τ PI for CMIN and CMAX). There is evidence elsewhere that optical dipole traps can lead to sub-Doppler atomic temperatures [15] , [16] . Systematic errors resulting from lattice intensity variations have essentially no effect on the ratios. With the overall good agreement between the measurement results and the model based on equation (1), we confirm that the photoionization process occurs close to the nucleus in the atom. Classically, the photoionization process occurs close to the nucleus because the Rydberg electron is able to exchange energy with the light field efficiently when it is undergoing maximal Coulomb acceleration at the inner turning point of its classical orbit. In contrast, when the Rydberg electron is far away from the nucleus, it behaves like a free electron, oscillating in a quiver motion at the frequency of the laser light although not exchanging energy with the light field. However, close to the nucleus, the Rydberg electron is strongly accelerated by the Coulomb field, and the electron is able to exchange energy with the light field by an amount proportional to its Coulomb acceleration squared [17] . From a quantum mechanical point of view, the photoionization process occurs close to the nucleus since the matrix element accumulates its value within a small volume near the nucleus. In Fig. 3a , we show how the calculated matrix element builds up as a function of cutoff radius for the dipole-allowed transition from to the continuum state as well as for the strongest dipole-violating transition from to . In the calculation, the photoionizing light field has a wavelength of 1,064 nm and is polarized in the z direction. The calculation is performed without making the dipole approximation (Methods). 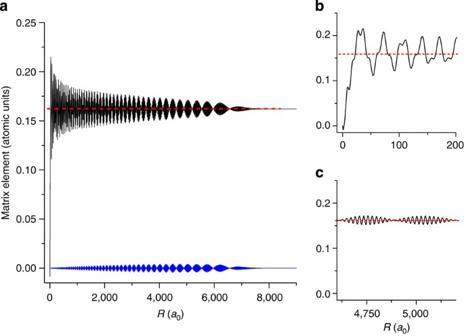Figure 3: Accumulation of the photoionization matrix element. (a) The value of the matrix element as a function of cutoff radiusRin the radial integration for transitions fromto(dipole-allowed, top) and to(dipole-violating, bottom). The field has a wavelength of 1,064 nm (ω=0.0428 atomic units). The matrix element for the dipole-violating transition is essentially zero. (b,c) The matrix element for the dipole-allowed transition accumulates to its asymptotic value (red dashed line) within a radius of ~50ao(b). The oscillations further out do not result in any additional accumulation (c). Figure 3: Accumulation of the photoionization matrix element. ( a ) The value of the matrix element as a function of cutoff radius R in the radial integration for transitions from to (dipole-allowed, top) and to (dipole-violating, bottom). The field has a wavelength of 1,064 nm ( ω =0.0428 atomic units). The matrix element for the dipole-violating transition is essentially zero. ( b , c ) The matrix element for the dipole-allowed transition accumulates to its asymptotic value (red dashed line) within a radius of ~50 a o ( b ). The oscillations further out do not result in any additional accumulation ( c ). Full size image For the dipole-allowed transition in Fig. 3 , the matrix element accumulates its value within a radius of about 50 a o from the nucleus, as highlighted in Fig. 3b , and then oscillates about its asymptotic value, a finding in accordance with calculations performed elsewhere [5] . There are two oscillation periods for radii larger than 50 a o , highlighted in Fig. 3c . The longer period is the deBroglie wavelength of the bound-state wavefunction (within its classically allowed regime), whereas the shorter period is that of the continuum state. The matrix element does not accumulate further for r ≳ 50 a o due to the large difference in the wavelengths of the bound and free states in this regime, leading to near-perfect cancellation in that integration domain. The radiative interaction is effectively confined to the region r ≲ 50 a o , where the deBroglie wavelengths are quite similar. As the region with r ≲ 50 a o is much smaller than the wavelength of the light, the dipole approximation is retroactively validated. It is therefore the light-field intensity at the nucleus of the atom that must be used in the calculation of the photoionization rates. The matrix element for the dipole-violating transition of Fig. 3a does not accumulate to any appreciable value in the domain r ≲ 50 a o and undergoes some oscillation about its near-zero asymptotic value in the domain r ≳ 50 a o . The photoionization probability for the dipole-violating case in Fig. 3a is only about 10 −6 times the dipole-allowed photoionization probability. Hence, the dipole approximation is very well satisfied. Atomic trajectories in the lattice We now adopt the fact that photoionization occurs near the nucleus and consider the Rydberg-atom trajectories in the lattice to explain several other trends in the data of Fig. 2c,d . During the 3 μs atom–field interaction time, the atoms move away from their initial positions on trajectories governed by the lattice adiabatic potentials V R ( Z )=( e 2 )/(2 mω 2 ε o c ) ∬ P ( z ) I ( z + Z ) d z (refs 14 , 18 ). As the electron density P ( z ) acts as a weighting factor, wavefunctions with larger spatial extents in the z direction usually result in more averaging and hence in shallower adiabatic potentials V R ( Z ) in the lattice. For the same n , level no. 2 atoms have larger spatial extents in z than level no. 5 atoms, generally resulting in shallower V R ( Z ). For most levels, the V R ( Z ) maxima coincide with lattice intensity maxima (non-flipped ‘NF’ case in Fig. 4a ). However, for ratios of atom size to lattice period near 1, the V R ( Z ) maxima coincide with lattice intensity minima (flipped ‘FL’ case in Fig. 4a ) [19] . As shown in Table 1 , the modulation depth of the V R ( Z ) generally decreases from level A to G. Atomic motion in shallower V R ( Z ) cause τ PI for CMIN and for CMAX to approach each other. Consequently, we observe a general drop in the ratios of Fig. 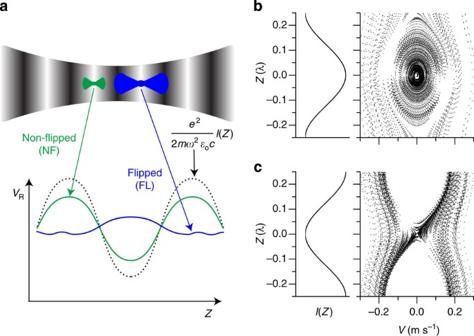Figure 4: Rydberg-atom trapping potentials and trajectories in an optical lattice. (a) Typical trapping potentialsVR(bottom) for the Rydberg wavefunctions (top) in the optical lattice (top, white indicates high intensity and black low intensity; bottom, intensityI(Z) is proportional to dotted line). Usually, potential maxima are co-located with intensity maxima (green). For wavefunctions with spatial extents in theZdirection slightly larger than the lattice period, potential maxima are ‘flipped’ (blue). (b,c) Simulated phase space diagrams (positionZversus velocityV) for the lattice-induced motion of level G atoms (which have flipped trapping potentials), with initial conditions CMAX (b) and CMIN (c), and correspondingI(Z). 2d from A to G. Figure 4: Rydberg-atom trapping potentials and trajectories in an optical lattice. ( a ) Typical trapping potentials V R (bottom) for the Rydberg wavefunctions (top) in the optical lattice (top, white indicates high intensity and black low intensity; bottom, intensity I ( Z ) is proportional to dotted line). Usually, potential maxima are co-located with intensity maxima (green). For wavefunctions with spatial extents in the Z direction slightly larger than the lattice period, potential maxima are ‘flipped’ (blue). ( b , c ) Simulated phase space diagrams (position Z versus velocity V ) for the lattice-induced motion of level G atoms (which have flipped trapping potentials), with initial conditions CMAX ( b ) and CMIN ( c ), and corresponding I ( Z ). Full size image The atomic trajectories in the lattice fall into four cases: atoms prepared with initial condition CMAX or CMIN, in either NF or FL potentials. In the CMAX/NF case ( Fig. 2c , squares, A–E), the atoms are initially prepared in regions of high intensity that are co-located with V R ( Z ) maxima. These atoms tend to quickly move through the lattice wells, sampling regions of both high and low intensity. Consequently, we expect these atoms to experience an average intensity at the nucleus given by I ( Z ) averaged over Z (in our experiment ~1.2 times the intensity of the ingoing lattice beam, independent of the level). The values in this case are therefore expected to be approximately the same for all tested levels, which we observe in Fig. 2c . In the CMAX/FL case ( Fig. 2c , squares, F and G), the atoms are initially prepared in regions of high intensity that are co-located with V R ( Z ) minima. Comparing the estimated initial kinetic energy of the atoms (~1.6 MHz) with the depth of the trapping potentials (1.1 and 3.1 MHz for F and G, respectively), we expect atoms in level G to be trapped at locations where the intensity at the atomic nucleus is high; this is illustrated in the phase space plot of Fig. 4b . We therefore expect level G to have one of the shortest , which is indeed observed. In the CMIN/NF case ( Fig. 2c , triangles, A–E), the atoms are initially prepared in regions of low intensity that are co-located with V R ( Z ) minima. For deep NF potentials (levels A–C; sixth column in Table 1 ), the atoms are strongly confined near the intensity minima and therefore have particularly long , as observed. For shallower potentials, the atoms are less strongly confined to the intensity minima, and consequently the observed drop somewhat. For the CMIN/FL case ( Fig. 2c , triangles, F and G), atoms sample all regions of the lattice fairly uniformly, as seen in Fig. 4c , and consequently have shorter (although still longer than in the CMAX/FL case, as for CMIN the atoms start at locations of low intensity). Deviations in the data from the general trends described above are the result of the systematic variations in day-to-day performance of the experiment discussed earlier, such as variations in lattice intensity and alignment. Using a spatially resolved light probe, we have provided direct experimental evidence that the photoionization of Rydberg atoms by light occurs close to the nucleus in an atom, a fundamental assumption underpinning experiments for decades. Photoionization rates measured for several Rydberg states depend on the light-field’s intensity near the centre of the atom, and not on the overlap of the electronic probability distribution with the light field. This result accords with the fact that the matrix element M r in equation (1) accumulates within a range that is small with respect to the impinging radiation. An essential experimental tool in our work has been an optical lattice, which enables spatially resolved photoionization. The storage and manipulation of Rydberg atoms in laser traps is important in several emerging areas, including the realization of exotic phases of matter [20] , field sensors [21] , quantum information processing [22] , [23] , [24] and high-precision measurements of fundamental constants [25] . In these applications, photoionization can either represent a mechanism through which Rydberg atoms are lost, or be exploited as a detection method [26] , [27] . Optical lattice The one-dimensional optical lattice is established by focusing a 1,064 nm beam (power 0.88–1.10 W) into a magneto-optical trap, retro-reflecting and refocusing it. The ingoing lattice beam is focused to a full-width at half-maximum (FWHM) of the intensity profile of 13 μm. The return beam has a FWHM of 25 μm, which is larger than the ingoing beam focus due to cumulative aberrations caused by the optical components in the retro-reflection beam path [28] . Also, the optical components in the beam path reduce the power of the return lattice beam at the location of the atoms to 0.56 times that of the ingoing beam. The reduction in power and enlargement in focus of the return beam means that the lattice is not a perfect standing wave; there is a running-wave component to the lattice. However, the intensity contrast between maxima and minima in the lattice is still about a factor of 5, allowing for a very clear distinction in the decay rates near these locations. The maximal lattice intensity is on the order of 10 8 W cm −2 . The lattice is linearly polarized in the x direction ( Fig. 1 ) and is always on for measurements involving the optical lattice. Excitation scheme Ground-state atoms are transferred to Rydberg states via two-photon excitation (excitation-pulse duration 0.5 μs). The lower-transition laser has a focus FWHM of 150 μm, a wavelength of 780 nm and a detuning of ≈1.2 GHz from the 5 P 3/2 intermediate state. The upper-transition laser has a focus FWHM of ~15 μm, has a wavelength of ≈480 nm and is tuned into two-photon resonance with a 5 S → nD transition (45≤ n ≤65). Control of the initial Rydberg-atom position To prepare the initial Rydberg-atom centre-of-mass positions near either intensity maxima or minima in the lattice, we use an electro-optic modulator to apply a controllable phase shift to the lattice’s return beam immediately following Rydberg excitation [28] . Ground-state atoms in our lattice are collected at intensity maxima as the lattice light is red-detuned relative to the 5 S →5 P transition of Rb. Therefore, with no phase shift applied after excitation to Rydberg states, the Rydberg-atom centre-of-mass positions are initially located near intensity maxima (CMAX). With a π phase shift applied to the return beam, the Rydberg-atom centre-of-mass positions are prepared near intensity minima in the lattice (CMIN). Photoionization calculation In the evaluation of equation (1), we sum σ PI over all allowed continuum states | f ›=| ε ′, l ′, j ′, m j ′›. The matrix elements M r =‹ f | x | i › are in atomic units, with the free wavefunctions normalized in unit energy, and are evaluated for | i › being the no. 2 or no. 5 Stark states. In the comparison model, the photoionization rate is proportional to ∬ P ( z ) I ( z + Z )d z and is normalized such that the two models have the same photoionization rate when averaged over one lattice period. In Fig. 3 , we use the formulation for the matrix elements , which does not include the electric dipole approximation and the light polarization is along z . In the calculations of M p as a function of cutoff radius R , we see that the matrix elements accumulate within ~50 a o from the nucleus, a distance much smaller than the light field’s wavelength. After having established that the approximation is exquisitely well satisfied, we use the simpler photoionization matrix element M r =‹ f | x | i › in equation (1), where the electric dipole approximation is implied and the light polarization is chosen along x . How to cite this article: Anderson, S. E. and Raithel, G. Ionization of Rydberg atoms by standing-wave light fields. Nat. Commun. 4:2967 doi: 10.1038/ncomms3967 (2013).